Fabrication of flexible and freestanding zinc chalcogenide single layers Inorganic graphene analogues (IGAs) are a conceptually new class of materials with attractive applications in next-generation flexible and transparent nanodevices. However, their species are only limited to layered compounds, and the difficulty in extension to non-layered compounds hampers their widespread applicability. Here we report the fabrication of large-area freestanding single layers of non-layered ZnSe with four-atomic thickness, using a strategy involving a lamellar hybrid intermediate. Their surface distortion, revealed by means of synchrotron radiation X-ray absorption fine structure spectroscopy, is shown to give rise to a unique electronic structure and an excellent structural stability, thus determining an enhanced solar water splitting efficiency and photostability. The ZnSe single layers exhibit a photocurrent density of 2.14 mA cm −2 at 0.72 V versus Ag/AgCl under 300 W Xe lamp irradiation, 195 times higher than that of bulk counterpart. This work opens the door for extending atomically thick IGAs to non-layered compounds and holds promise for a wealth of innovative applications. Two-dimensional (2D) nanomaterials such as graphene are a conceptually new class of materials that offer new opportunities for high-quality and large-area nanodevices [1] , [2] . Beyond graphene itself, inorganic graphene analogues (IGAs) with high percentage of surface atoms have recently sparked worldwide interests owing to their novel properties and great potential for applications in transistors [2] , energy storage [3] , [4] , thermal conductors [5] and topological insulators [6] . Although the IGAs often bring on a wealth of innovative applications, their species are still only limited to layered compounds. In other words, controllable exfoliation of layered compounds is regarded as the exclusive way to obtain single-layered IGAs with few atomic thickness [7] , [8] , [9] , whereas the hard bond-cleavage of non-layered compounds enables the fabrication of their single layers with few atomic thickness become a great challenge. Despite recent progress in fabricating CdSe 2D sheets with few atomic thickness [10] , [11] , the difficulties in the removal of nonvolatile organic solvents and the occurrence of aggregation during slow solvent evaporation unfortunately bring difficulty to process them into devices [12] . This raises some important questions. For example, how can one develop a universal strategy for fabricating clean single layers of non-layered compounds with few atomic thickness? How can the clean single layers of non-layered compounds be stable at ambient conditions? Can the clean and freestanding single layers of non-layered compounds with few atomic thickness bring unprecedented properties? In this regard, some natural phenomena give us important inspirations: a batch of papers naturally separate into many pieces of paper or a shale is easily split into many thin flakes under the effect of external forces. The study of these natural phenomena reminds us that lamellar hybrid structures may become a bridge between initial non-layered compounds and final graphene-like single layers with few atomic thickness. Here, taking the non-layered zinc chalcogenides ZnSe and ZnS with zinc-blende structure as examples, we develop a versatile and scalable lamellar hybrid intermediate strategy for synthesizing clean and freestanding single layers of non-layered compound with few atomic thickness. Characterizations of freestanding ZnSe single layers Our method is summarized in Fig. 1a . Taking zinc chalcogenide ZnSe as an example ( Supplementary Fig. S1 ), clean and freestanding ultraflexible ZnSe single layers with four-atomic thickness were first successfully synthesized by virtue of lamellar hybrid (Zn 2 Se 2 )(pa) (pa stands for n -propylamine) intermediate, in which hybrid ZnSe-pa single layers were initially exfoliated and then pa molecules were removed by heat treatment at 140 °C for 2 h ( Supplementary Fig. S2 ). The colloidal suspension of clean ZnSe single layers was highly stable over several days and displayed Tyndall phenomenon, reasonably inferring the formation of stable and homogeneous ZnSe single layers ( Fig. 1b and Supplementary Fig. S3 ) [13] . Transmission electron microscopic (TEM) image in Fig. 1b further illustrated their uniform freestanding and large-area sheet-like morphology with lateral size of ca 500 nm, whereas the inset high-magnified TEM image clearly revealed their highly flexible and nearly transparent features. Atomic force microscopic image in Fig. 1c and Supplementary Fig. S4 clearly showed the extremely smooth and large 2D sheets with an average height of 0.91 nm, matching well with the 0.85 nm thickness for single-layer [Zn 2 Se 2 ] slab in the lamellar (Zn 2 Se 2 )(pa) intermediate [14] , which provided a direct and reliable evidence for the formation of large-area ZnSe single layers with four-atomic thickness ( Supplementary Fig. S2 ). In addition, X-ray photoelectron spectroscopy, Fourier transform infrared spectrum and thermogravimetric analysis in Supplementary Figs S5 and S6 demonstrated the absence of pa molecules, giving direct evidence for the formation of clean ZnSe single layers. Moreover, X-ray diffraction pattern in Fig. 1e clearly revealed that the ZnSe single layers possessed a highly (110) preferred orientation, further verified by their corresponding high-resolution TEM image and fast Fourier transform image in Fig. 1d . Of note, as for II–VI semiconductor compounds such as zinc-blende ZnSe, structural analysis reveals that the (110) facets are their cleavage and nonpolar planes [15] . As such, the zinc-blende ZnSe could be relatively easily cleaved along the (110) plane under certain forces, whereas the exposed neutral (110) facet could render it much more stable than other exposed polar planes such as (100) or (111) facet, which can be further validated by the corresponding calculated surface energies in Supplementary Methods and Supplementary Figs S7 and S8 . 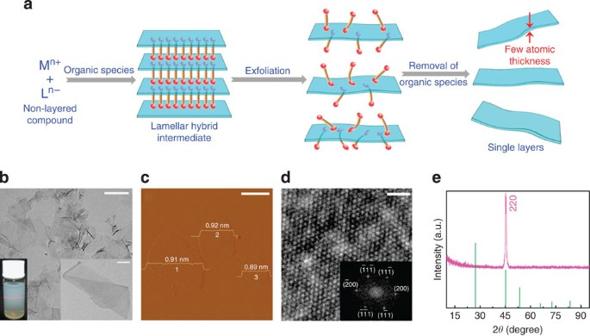Figure 1: General synthetic strategy and characterizations of ZnSe freestanding single layers. (a) A general lamellar hybrid intermediate strategy for synthesizing clean and freestanding single layers of non-layered compound with few atomic thickness; characterizations for large-area flexible ZnSe freestanding single layers. (b) TEM images and the corresponding colloidal ethanol dispersion displaying Tyndall effect, scale bar, 500 nm and the inset scale bar, 100 nm. (c) Atomic force microscopic image with an average thickness of 0.91 nm, scale bar, 500 nm. (d) HRTEM and the corresponding fast Fourier transform, scale bar, 1 nm. (e) XRD pattern, the olive lines give the corresponding standard pattern of JCPDS card no. 88-2345. Figure 1: General synthetic strategy and characterizations of ZnSe freestanding single layers. ( a ) A general lamellar hybrid intermediate strategy for synthesizing clean and freestanding single layers of non-layered compound with few atomic thickness; characterizations for large-area flexible ZnSe freestanding single layers. ( b ) TEM images and the corresponding colloidal ethanol dispersion displaying Tyndall effect, scale bar, 500 nm and the inset scale bar, 100 nm. ( c ) Atomic force microscopic image with an average thickness of 0.91 nm, scale bar, 500 nm. ( d ) HRTEM and the corresponding fast Fourier transform, scale bar, 1 nm. ( e ) XRD pattern, the olive lines give the corresponding standard pattern of JCPDS card no. 88-2345. Full size image Synchrotron X-ray absorption fine structure measurements It is well known that the X-ray absorption fine structure (XAFS) is a powerful element-specific tool to study local atomic arrangements and electronic structures of condensed matters. To interpret the stability of clean ZnSe single layers with four-atomic thickness, we performed synchrotron radiation XAFS measurements at both Zn and Se K -edges. The Zn K -edge k χ( k ) oscillation curves in Fig. 2a exhibited remarkable differences among bulk ZnSe, exfoliated ZnSe-pa single layers and clean ZnSe single layers, especially in the 2−6 Å −1 k -region, implying the different local atomic arrangement of clean ZnSe single layers with their bulk counterpart and exfoliated ZnSe-pa single layers. These differences could be more explicitly manifested by the R -space curves as shown in Fig. 2b . The Fourier transforming curves of bulk ZnSe were characterized by two main peaks at 2.11 and 3.63 Å, corresponding to the nearest Zn–Se and next nearest Zn–Zn coordinations, respectively. For the exfoliated ZnSe-pa single layers, the intensities of these two peaks decreased significantly, associated with noticeable shift of the Zn–Zn peak position to 3.52 Å. At the same time, a new peak at 1.57 Å appeared, confirming the presence of pa molecules. Contrastingly, for the final clean ZnSe single layers, the Zn–Se peak was shifted to 2.17 Å along with a decrease in peak intensity and the Zn–Zn peak became very weak, and most importantly, the peak at 1.57 Å disappeared again, demonstrating the successful removal of pa molecules. Of note, the above Zn K -edge data for clean ZnSe single layers qualitatively revealed their distinct local atomic arrangement compared with ZnSe-pa single layers and bulk counterpart, which could be further verified by their Se K -edge data, that is, the Se–Se peak position was shifted to higher- R side and the peak intensity was greatly reduced for the exfoliated ZnSe-pa single layers and clean ZnSe single layers with regard to bulk ZnSe ( Fig. 2a,b ). 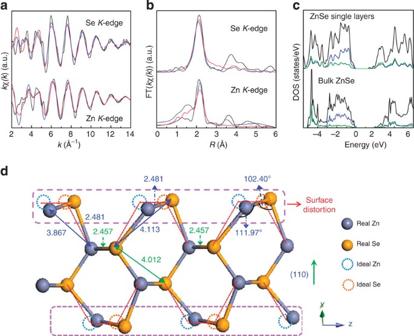Figure 2: Synchrotron radiation XAFS measurements and calculated DOS. (a) Zn and SeK-edge extended XAFS oscillation functionkχ(k) and (b) the corresponding Fourier transforms; the red, blue and black lines correspond to ZnSe single layers, ZnSe-pa single layers and bulk ZnSe, respectively; (c) the calculated DOS, the black, blue and olive lines denote the total, Se sp and Zn sp state density, respectively; ZnSe single layers and bulk ZnSe had calculated band gaps of 1.25 and 1.07 eV, respectively; (d) structural model of ZnSe single layers viewed along the (110) plane. Figure 2: Synchrotron radiation XAFS measurements and calculated DOS. ( a ) Zn and Se K -edge extended XAFS oscillation function k χ( k ) and ( b ) the corresponding Fourier transforms; the red, blue and black lines correspond to ZnSe single layers, ZnSe-pa single layers and bulk ZnSe, respectively; ( c ) the calculated DOS, the black, blue and olive lines denote the total, Se sp and Zn sp state density, respectively; ZnSe single layers and bulk ZnSe had calculated band gaps of 1.25 and 1.07 eV, respectively; ( d ) structural model of ZnSe single layers viewed along the (110) plane. Full size image The high-quality extended XAFS spectra enabled us to further perform least-squares fittings for the Zn and Se K -edge data, and the obtained quantitative results were summarized in Supplementary Table S1 and Supplementary Fig. S9 . The most important results as revealed from Supplementary Table S1 were that the coordination between Zn atoms and pa molecules resulted in slight expansion of the surface Zn–Se bond lengths, but the next nearest Zn–Zn distances (3.85 Å) were contracted and the Se–Se distances (4.11 Å) were elongated considerably, as compared with the bulk value (4.012 Å). This meant a noticeable distortion on the surface of exfoliated ZnSe-pa single layers, and these clean ZnSe single layers still preserved the surface distortion that in turn helped to decrease their surface energy and then endow them with excellent stability [16] . Thus, the surface distortion associated with the high (110)-orientation synergistically ensured the high structural stability of these clean ZnSe single layers. From the structural parameters of Supplementary Table S1 obtained by XAFS, we depicted the structure model of the ZnSe single layers in Fig. 2d in which the distorted bond lengths and bond angles were clearly labelled. As a result of the expanded nearest Zn–Se bond length and contracted next nearest Zn–Zn distance, the surface Zn–Se–Zn bond angle of ZnSe single layers exhibited a significant compression of 7.0° from the bulk value of 109.5°. On the contrary, their surface Se–Zn–Se bond angle was stretched by an amount of 2.5°. Undoubtedly, the surface distortion of ZnSe single layers would significantly influence their electronic properties, and therefore, density functional theory calculations were performed based on the atomic structural parameters by XAFS. The obtained densities of states (DOS) for ZnSe single layers and bulk ZnSe were displayed in Fig. 2c . The DOS of bulk ZnSe exhibited a low tail at the conduction band minimum, whereas the ZnSe single layers displayed obviously raised states density at the edge of conduction band. This greatly increased DOS at the conduction band minimum of the ZnSe single layers could be ascribed to their exotic single-layered structure with obvious surface distortion. As the separation and transportation ability of electron is positively related to density of states of the band edge [17] , it can be declared that the larger states density of conduction band edge of ZnSe single layers ensures a high migration rate and overcomes the shortcoming of bulk ZnSe, thus contributing to their excellent electronic properties. As a result, the synchrotron radiation XAFS and first-principles calculation reveal that the surface distortion endows ZnSe single layers with excellent structural stability and unique electronic structure, thus providing the prerequisites for realizing their strong photostability and high-photocurrent density. Also, it should be noted that, at ambient conditions, a small amount of water, CO 2 , O 2 or so on may be physically adsorbed on the surface of ZnSe single layers to further ensure their high stability, while these adsorbed species did not change their surface structure, which could be verified by the corresponding XAFS measurements in Fig. 2a,b . A general and scalable strategy Of note, the strategy for synthesizing large-area flexible ZnSe freestanding single layers with high transparency is not limited to ethanol but can be extended to a wide range of other solvents, such as butanol, dodecanol, isopropanol, 1,4-butylene glycol, 1,3-butylene glycol, nucleoside 5′-phosphate and dimethyl sulphoxide ( Supplementary Fig. S10 ). Note that most of the above solvents possessed low-boiling points, which could offer several obvious advantages, such as easy removal, low cost, lower toxicity and better biocompatibility [18] . In addition, to deeply understand the exfoliation process, we also achieved ZnSe-pa sheets with a desired number of layers through controlling the sonication time of (Zn 2 Se 2 )(pa) in ethanol ( Supplementary Figs S11–S13 ). Moreover, to further verify the generality of this lamellar hybrid intermediate strategy, we synthesized other large-area flexible and freestanding single layers of non-layered zinc-blende ZnS ( Supplementary Fig. S14 ). Thus, this developed strategy is general and may be extended to the vast majority of non-layered compounds. Also, this approach is quick, simple and can be easily scaled up, as the throughput is only limited by the size of vessel. Photoelectrochemical properties Of note, just as the graphene displayed peculiar electronic properties when fabricated into flexible and transparent devices [19] , [20] , the large-area zinc chalcogenide single layers with few atomic thickness may also exhibit a wealth of innovative properties. Here, we highlight the first discovered and preliminary results as the ultraflexible and transparent photoelectrode in photoelectrochemical (PEC) solar water splitting, which will definitely make semiconductor single layers with few atomic thickness as the new spotlight in solar water splitting field. As is well known, solar water splitting can overcome the limited supply of fossil fuels and greenhouse effect, but the low efficiency and poor material stability impede its practical applications. As such, it is urgent to pursue an appropriate material system in efforts to achieve highly efficient PEC properties. Notably, the direct semiconductor behaviour associated with high carrier mobility of 1,250 cm 2 V −1 s −1 makes the environmentally benign ZnSe very attractive for constructing optoelectronic devices [14] , [21] . Thus, the photoelectrodes of ZnSe thin films were prepared by spin coating the corresponding ethanol dispersions for testing their water photoelectrolysis properties. As depicted by Supplementary Fig. S15A , the ZnSe single layers with four-atomic thickness displayed almost completely transparent, whereas other films gradually changed to grey with the increasing layers of ZnSe sheets, and their bulk counterpart is of yellow opacity, matching well with the ultraviolet–visible analysis results in Supplementary Fig. S15B in which one can clearly see that the ZnSe single layers only absorbed ultraviolet light compared with the bulk counterpart. The water photoelectrolysis properties of ZnSe films were first investigated by the photocurrent measurements in a 0.5 M Na 2 SO 4 electrolyte using a three-electrode setup. 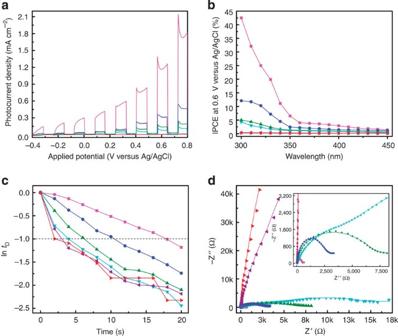Figure 3: Photoelectrochemical properties. (a) Photocurrent density versus applied potential curves under chopped 300 W Xe lamp irradiation; (b) IPCE; (c) transient decay time and (d) electrochemical impedance spectra at 0.6 V versus Ag/AgCl under 300 W Xe lamp irradiation; the magenta, blue, olive, cyan, purple and red plots correspond to ZnSe single layers, ZnSe-pa double layers and quadruple layers, ZnSe-pa octuple layers, (Zn2Se2)(pa) and bulk ZnSe, respectively; Z′ and Z″ indare the real and imaginary parts of impedance, whereas the solid lines are fitted by ZSimpWin software using the equivalent circuits. Figure 3a revealed that the dark current of all ZnSe films remained a very low level (<5 μA cm −2 ) under applied potentials between −0.4 and 0.8 V. On the irradiation of 300 W Xe lamp containing only ca 4% ultraviolet spectrum, the ZnSe single layers exhibited a much pronounced photocurrent density of 2.14 mA cm −2 at 0.72 V versus Ag/AgCl, roughly 195 times higher than their bulk counterpart. Contrastingly, the ZnSe-pa double layers, quadruple layers and octuple layers displayed 49, 24 and 14 times higher photocurrents than the bulk counterpart. Also, Supplementary Fig. S16 clearly revealed that the ZnSe single layers exhibited strong intensity and frequency-dependent photocurrent densities, and also possessed significantly higher photocurrent densities than all the other ZnSe samples. As shown in Supplementary Fig. S17 , one can clearly observe that the ZnSe single layers achieved a roughly eight times higher photocurrent density than that of the clean ZnSe quantum-dots with an average size of ca 3–4 nm at 0.72 V versus Ag/AgCl, further demonstrating their remarkably efficient PEC water splitting. Figure 3: Photoelectrochemical properties. ( a ) Photocurrent density versus applied potential curves under chopped 300 W Xe lamp irradiation; ( b ) IPCE; ( c ) transient decay time and ( d ) electrochemical impedance spectra at 0.6 V versus Ag/AgCl under 300 W Xe lamp irradiation; the magenta, blue, olive, cyan, purple and red plots correspond to ZnSe single layers, ZnSe-pa double layers and quadruple layers, ZnSe-pa octuple layers, (Zn 2 Se 2 )(pa) and bulk ZnSe, respectively; Z′ and Z″ in d are the real and imaginary parts of impedance, whereas the solid lines are fitted by ZSimpWin software using the equivalent circuits. Full size image Moreover, the incident photon-to-current conversion efficiency (IPCE) onset of ZnSe single layers was at around 350 nm ( Fig. 3b ), which corresponded to a 3.5 eV band-gap, fitting well with their measured absorption edge in Supplementary Fig. S15A . Intriguingly, Fig. 3b clearly validated their highest IPCE of 42.5% at 300 nm, which was strikingly higher than that of bulk ZnSe (0.25%), (Zn 2 Se 2 )(pa) (0.4%), ZnSe-pa octuple layers (4.3%), ZnSe-pa quadruple layers (5%) and ZnSe-pa double layers (12.1%). To the best of our knowledge, the photoconversion efficiency of 42.5% is much better than that of most existing reports [22] , [23] . This extraordinary IPCE of the ZnSe single layers could be attributed to their several clear-cut advantages including ultraflexible, large-area, atomic thickness and high (110) orientation, which would be detailedly discussed below. Moreover, compared with the striking colour change and large I - t fluctuations occurred in bulk ZnSe ( Supplementary Fig. S18 ), the ZnSe single layers displayed negligible variations after even 3,600 s irradiation, revealing their much better photostability, which was further verified by their highly reproducible I - t curves in Supplementary Fig. S15C . It was notable that their excellent photostability benefited from their strong structural stability. The decreasing photocurrents of each light on cycle in Supplementary Fig. S15C indicated the recombination of charge carriers within the films [21] . To further study their charge recombination behaviour, the transient decay time was calculated according to the following formula: where I in and I t stand for the photocurrent density at 0 s and t s, I st represents the steady-state photocurrent density ( Supplementary Fig. S15D ). The transient time constant of τ is defined as the decay time when ln t D =−1 (ref. 24 ). ZnSe single layers showed a τ up to 18.1 s in Fig. 3c , prominently higher than that of bulk ZnSe (1.9 s), (Zn 2 Se 2 )(pa) (3.0 s), ZnSe-pa octuple layers (3.9 s), ZnSe-pa quadruple layers (6.2 s) and ZnSe-pa double layers (10.4 s), implying the much slower charge recombination process for ZnSe single layers. Accordingly, for the ZnSe single layers, their eminently larger photocurrent density, remarkably higher IPCE and much better photostability could be ascribed to the synergistic effect between their macroscopic morphological features and microscopic electronic structure. The huge specific surface area and high percentage of distorted surface atoms enabled them to harvest greatly increased ultraviolet light ( Supplementary Fig. S15B ) [25] , whereas obvious light transmittance and reflection usually occur in bulk particles ( Fig. 4 ). Also, according to the diffusion formula of t = d 2 / k 2 D ( d is the particle size, k is a constant, D is the diffusion coefficient of electron-hole pairs) [26] , their unique electronic structure ( Fig. 2c ) associated with atomically ultrathin thickness and high (110)-orientation could endow them with unusual electronic properties including higher carrier mobility and better grain boundary connectivity [27] , [28] , verified by their corresponding charge transfer resistance in Fig. 3d . The ZnSe single layers with four atomic thickness exhibited the lowest charge transfer resistance, helping to achieve highly efficient carrier transport and separation efficiency as well as low corrosion rates. Note that the low corrosion rates, the high (110)-orientation and the obvious surface distortion synergistically rendered them high photostability. Obviously, their ultraflexible features could achieve an intimate contact with the indium tin oxide (ITO) substrate, hence, facilitating electrons to effectively circulate through the external circuit. Moreover, benefited from a larger contact area with electrolyte, the ZnSe single layers allowed surface reactions to take place across a much bigger area, greatly enlarging the reaction space [29] . By contrast, as for bulk counterpart, the large and irregular shapes result in many grain boundaries and poor contact with substrate, which leads photoexcited electrons to diffuse through countless recombination centres before reaching the photoelectrodes, thus causing loss of the vast majority of those charge carriers. Furthermore, Fig. 3a,d also demonstrated that the presence of pa molecules limited the efficient carrier transport through ZnSe layers and then decreased their PEC properties [30] , further verifying the charming superiority of clean single layers as the high-performance PEC photoelectrodes. 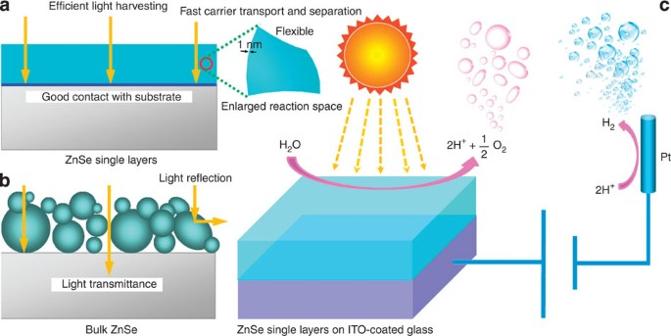Figure 4: Advantages of single-layer ZnSe-based film photoelectrode. (a,b) Advantages of using large-area flexible ZnSe freestanding single layers versus bulk ZnSe deposited on indium tin oxide (ITO)-coated glass as the photoelectrodes for solar water splitting. (c) Working mechanism of a PEC device for solar hydrogen production using ZnSe single layers as the photoanode. Figure 4: Advantages of single-layer ZnSe-based film photoelectrode. ( a , b ) Advantages of using large-area flexible ZnSe freestanding single layers versus bulk ZnSe deposited on indium tin oxide (ITO)-coated glass as the photoelectrodes for solar water splitting. ( c ) Working mechanism of a PEC device for solar hydrogen production using ZnSe single layers as the photoanode. Full size image To summarize, we have fabricated large-area flexible ZnSe freestanding single layers with four-atomic thickness. Their surface distortion, revealed by synchrotron radiation XAFS, is shown to endow them with a unique electronic structure and excellent structural stability, thus determining their enhanced photoconversion efficiency and photostability. These ZnSe single layers exhibit a photocurrent density up to 2.14 mA cm −2 , 195 times higher than that of the bulk counterpart. Also, they display a pronounced IPCE of 42.5%, strikingly higher than that of the bulk counterpart (0.25%). The superior solar water splitting of ZnSe single layers with four-atomic thickness is undoubtedly only one of their many properties, leaving others to be explored. Meanwhile, this scalable lamellar hybrid intermediate strategy is expected to fabricate IGAs of all the other non-layered compounds, which will greatly expand the species of IGAs, thus opening new avenues for bringing on series of unprecedented excellent properties. Materials Commercially available zinc-blende ZnSe powders were purchased from Aldrich. In addition, hybrid (Zn 2 Se 2 )(pa) products were prepared according to literature [14] . Here, pa in the hybrid (Zn 2 Se 2 )(pa) stands for n -propylamine. In other words, the (Zn 2 Se 2 )(pa) hybrid is consisted of single-layer (Zn 2 Se 2 ) slabs regularly separated from each other by pa molecules. Synthesis of ZnSe single layers In a typical procedure, 40 mg (Zn 2 Se 2 )(pa) products and 40 ml ethanol were added into a weighing bottle with a capacity of 50 ml. The weighing bottle was then sealed with a rubber stopper and sonicated at a low-power sonic bath (KQ3200DA) for 4 h. The resultant dispersions were centrifuged at 500 r.p.m. for 40 min. After centrifugation, the dispersions become almost transparent; the supernatant (top four-fifth of the centrifuged dispersion) was collected by pipette. We estimated the mass remaining in the supernatant by drying and weighing the sediments in the centrifugal tube and found that about one-third of the starting material remained in the supernatant. In other words, the finally obtained colloidal supernatant possessed a concentration as high as 0.3 mg ml −1 . After heating the supernatant at 140 °C for 2 h with a view to volatilize the solvent and pa molecules, the final product of clean ZnSe single layers was collected for further characterization. Characterization XRD patterns were recorded by using a Philips X'Pert Pro Super diffractometer (Philips) with Cu Kα radiation ( λ =1.54178 ˚). TEM images and high-resolution TEM image were obtained by using a JEOL-2010 TEM with an acceleration voltage of 200 kV. The field emission scanning electron microscopic (SEM) images were obtained by using a FEI Sirion-200 SEM. X-ray photoelectron spectra were acquired on an ESCALAB MKII with Mg Kα (hυ=1253.6 eV) as the excitation source. The binding energies obtained in the X-ray photoelectron spectral analysis were corrected for specimen charging by referencing C 1 s to 284.5 eV. Atomic force microscopicstudy in the present work was performed by means of Veeco DI Nano-scope MultiMode V system. The infrared spectra were measured on a NICOLET Fourier transform infrared spectrometer, using pressed KBr tablets. Thermal gravimetric analysis of the as-synthesized samples was carried out on a Shimadzu TA-50 thermal analyzer (Shimadzu) at a heating rate of 5 °C min −1 from room temperature to 500 °C. The Zn K -edge and Se K -edge XAFS were measured at the 1W1B beamline of Beijing Synchrotron Radiation Factory (BSRF) and the U7C beamline of the National Synchrotron Radiation Laboratory (NSRL), China. The storage ring of the BSRF was operated at 2.5 GeV with a maximum current of 250 mA, and NSRL was operated with a storage ring working at the energy of 800 MeV and a maximum electron current of 300 mA. Room-temperature ultraviolet–visible diffuse reectance spectroscopy and ultraviolet–visible absorption spectra were recorded on a Perkin-Elmer Lambda 950 UV/Vis-NIR spectrophotometer (Perkin-Elmer). PEC measurement To conduct the PEC water splitting measurements, the ZnSe products were needed to be fabricated into films. The detailed fabrication process of the films was shown as follows: the ZnSe products were initially dispersed in the solvent of ethanol to obtain a concentration of 0.3 mg ml −1 ; then 5 ml ethanol dispersion of the above different structured ZnSe products was uniformly spin-dropped on the 1.5×2 cm 2 ITO-coated glass at 500 r.p.m. for 30 s by a desktop spin coater (KW-4A, made by the Chinese Academy of Sciences); afterwards, the ITO-coated glasses were heated at 60 °C for 30 min with a view to volatilize the solvent and then the films for different structured ZnSe were obtained for further measurements. PEC tests were carried out in a conventional three-electrode, single-compartment quartz cell filled with 0.5 M Na 2 SO 4 electrolyte (pH=6.6). The Na 2 SO 4 electrolyte was purged with nitrogen for 30 min before the measurement. The different structured ZnSe deposited on ITO-coated glass electrodes served as the working electrodes. The counter and the reference electrodes were the platinum gauze and the Ag/AgCl reference electrode, respectively. The PEC properties were measured on an electrochemical station (Zahner IM6ex, Germany) in ambient conditions under irradiation of a 300 W Xe lamp (PLS-SXE300/300UV, Trusttech, Beijing). The power density of light source used in the measurement is 50 mW cm −2 . The potential was swept from −0.4 to +0.8 V (versus Ag/AgCl) at a sweep rate of 10 mV s −1 . IPCE spectra were measured on a QE/IPCE Measurement Kit (Newport, USA), whereas all the kit components were in control of Oriel Tracq Basic V5.0 software automatically. The light from a 300-W Xe lamp was focused through a monochromator (74125 Oriel Cornerstone 260 1/4 m) onto the cell, and the monochromator was incremented through the spectral range (300–450 nm) to generate a photocurrent action spectrum with a sampling interval of 10 nm and a current sampling time of 2 s, where the light intensity and the photocurrent generated were measured with a 2931-C dual channel power/current metre and a 71675 calibrated ultraviolet silicon photodetector. IPCE can be expressed concretely as follows: where h is the Planck's constant, c is the speed of light, I is the measured photocurrent density at a specific wavelength, λ is the incident light wavelength and J light is the recorded irradiance intensity at a specific wavelength. The electrochemical impedance spectroscopy was performed on an electrochemical station (Zahner IM6ex, Germany) in 0.5 M Na 2 SO 4 electrolyte. The Nyquist plots were measured at a bias potential of 0.6 V versus Ag/AgCl with a frequency of 100 kHz–100 mHz under irradiation of a 300-W Xe lamp. The measured spectra were fitted by the ZSimpWin program (from Echem software). How to cite this article: Sun, Y. et al . Fabrication of flexible and freestanding zinc chalcogenide single layers. Nat. Commun. 3:1057 doi: 10.1038/ncomms2066 (2012).